Selective and mild hydrogen production using water and formaldehyde With the increased efforts in finding new energy storage systems for mobile and stationary applications, an intensively studied fuel molecule is dihydrogen owing to its energy content, and the possibility to store it in the form of hydridic and protic hydrogen, for example, in liquid organic hydrogen carriers. Here we show that water in the presence of paraformaldehyde or formaldehyde is suitable for molecular hydrogen storage, as these molecules form stable methanediol, which can be easily and selectively dehydrogenated forming hydrogen and carbon dioxide. In this system, both molecules are hydrogen sources, yielding a theoretical weight efficiency of 8.4% assuming one equivalent of water and one equivalent of formaldehyde. Thus it is potentially higher than formic acid (4.4 wt%), as even when technical aqueous formaldehyde (37 wt%) is used, the diluted methanediol solution has an efficiency of 5.0 wt%. The hydrogen can be efficiently generated in the presence of air using a ruthenium catalyst at low temperature. A major challenge in chemical science nowadays is to discover new approaches resolving the worldwide demands regarding more efficient energy storage systems. One promising solution involves hydrogen as an alternative energy carrier and feedstock for environmental and economic reasons. In particular, hydrogen storage is of great interest in combination with direct hydrogen fuel cells as efficient energy conversion systems [1] , [2] , [3] . The competitiveness of hydrogen and its superior energetic properties (123 MJ kg −1 ) in comparison with fossil fuels (diesel: 46 MJ kg −1 ) is still restricted owing to delivery problems. In particular, physical options such as high pressure and cryogenic storage suffer from the containers’ heavy weight and safety problems [4] . Therefore, one alternative is chemical hydrogen storage in molecular materials in which the dihydrogen is stored in the form of hydridic and protic hydrogen. Examples are metal hydrides [4] , [5] , [6] , ammonia borane derivatives [2] , [3] , [7] , formic acid [2] , [8] , [9] , [10] , [11] , [12] , [13] , [14] , [15] , [16] , [17] and methanol [18] , [19] , [20] , [21] . Ammonia borane derivatives have a good weight efficiency (≤19.4 wt% H 2 ) [2] , [3] , [7] , but the solid spent-fuels are hardly recyclable. Formic acid-based systems are robust [8] , [15] , [16] , but the H 2 weight efficiency is quite low (4.4 wt% H 2 ), and so far low-temperature methanol-based systems (12.5 wt% H 2 ) [18] are limited to inert conditions, as the nature of the catalysts is sensitive to air and might decompose under oxidative conditions. Moreover, the formic acid and methanol dehydrogenation require additional base, which is a drawback for the weight efficiency. Water (11 wt% H 2 ) as a sole source of hydrogen is desirable as it is cheap and readily available, but so far water-splitting schemes need large amounts of energy for the electrochemical, photolytic or thermal process [22] , [23] . Also, homogeneous water-splitting is rare and so not yet very suitable for application in terms of efficiency and significant hydrogen yields [24] . Formic acid and methanol have the advantages that only gaseous products (H 2 /CO 2 ) are formed, and in presence of molecular ruthenium catalysts no relevant CO and methane formation occurs [8] , [16] , [18] . In addition, these factors are crucial for mobile applications with hydrogen fuel cells where the formation of solid and liquid by-products as well as CO as a catalyst poison are detrimental for fuel cell catalysts. In our research on molecular hydrogen storage systems, we focus on low-temperature (40–140 °C; 313–413 K) hydrogen generation with non-inflammable compound mixtures with weight efficiencies of 4–13 wt% H 2 (refs 7 , 8 , 25 , 26 ). Interestingly, early reports about hydrogen production using methanol [20] or formic acid [17] go back to the early 1960s, but homogeneous-catalysed formaldehyde (FA)-assisted water-splitting has not been reported, to the best of our knowledge, in the last 5 decades. Moreover, the ‘renaissance’ for formic acid-based catalytic hydrogen production started only in 2008 (refs 15 , 16 ). Most recently, in 2013, homogeneous methanol reforming under basic conditions has been reported for the first time [18] . However, methanol steam reforming is well known with solid phase catalysts at high temperatures [21] , [27] , [28] , [29] , [30] , [31] , [32] , [33] , and intensively investigated with copper and zinc oxide catalysts [27] , [28] , [29] , [31] , [32] . Here we report a one-pot process with two dehydrogenation steps in aqueous media containing FA, where water acts as a hydrogen source as well. In the present work, we show that paraformaldehyde (pFA) and FA together with water are suitable materials for catalytic hydrogen production with defined selectivity and tolerance to oxygen-containing atmosphere. The process solely gives good yields of hydrogen and carbon dioxide in pure form. Owing to the long-term stability/recyclability, non-flammability and a theoretical H 2 weight efficiency of 8.4 wt%, considering 1 eq. H 2 O and H 2 CO forming stable methanediol ( vide infra ), this molecule is potentially interesting for mobile applications. The hydrogen content of methanediol is still higher than formic acid (4.4 wt%), even when technical aqueous FA (37 wt%) is used. Such diluted methanediol solution has a minimum efficiency of 5.0 wt%. Taking into account that the hydrogen from FA-assisted water-splitting can be used for fuel cells, it is advantageous that the oxygen, which is formally formed during a direct water-splitting reaction, is trapped simultaneously in the form of carbon dioxide. Consequently, the oxygen is not available for oxidation, avoiding deactivation/oxidation of the fuel cell catalyst. Moreover, the formation of explosive mixtures of hydrogen and oxygen gas (oxyhydrogen) is avoided and hydrogen is generated in a non-flammable liquid, which is safer than the application of methanol systems. Besides, mixtures of hydrogen and carbon dioxide are easier to handle and to separate than an oxyhydrogen gas mixture (H 2 /O 2 ). All these aspects make the FA-assisted water-splitting interesting for hydrogen production and complementary to the proposed methanol economy [21] , [33] . In addition, this catalytic conversion of aqueous FA might be an interesting approach for decontamination treatment of wastewater containing FA impurities, which can be easily converted into carbon dioxide and hydrogen. Beyond that, another potential application of this system is that the produced hydrogen can be used directly in transfer-hydrogenation reactions in organic synthesis. In the following, we describe the formation of hydrogen from aqueous FA and pFA, the composition of the gaseous and liquid phase in this process with isotopically labelled substrates, characterization of the catalyst species and the catalyst performance and its isolation. Methanediol formation and dehydrogenation The low-temperature reforming of pFA and FA in aqueous solution is catalysed by the commercially available [(Ru(p-cymene)) 2 ( μ -Cl) 2 Cl 2 ] 1 as the catalyst precursor, which was previously investigated in-depth for the decomposition of formic acid [8] . Contrary to the formic acid decomposition, no catalyst preactivation with base is needed for the pFA/FA decomposition. In water, it is known that FA is in principal solely present in the hydrated form as methanediol [34] , [35] . The equilibrium constant for methanediol/FA is K c =2 × 10 [3] in contrast to K c =2 × 10 −3 for 2,2-dihydroxypropane/acetone [34] , [35] . Therefore, hydrated FA makes water accessible for dehydrogenation in aqueous solution, where methanediol acts as the hydrogen source. Thus, in the homogeneous processing of methanol or FA in an aqueous dehydrogenation reaction to CO 2 and H 2 , it is more likely that the coordinated methanediol plays a role rather than the side-on coordination of the FA as proposed elsewhere [18] . Considering that FA is produced by methanol oxidation (Formox process) with water as a by-product, the protic hydrogen atoms in methanediol are originally derived from methanol due to hydrolysis of FA ( Supplementary Fig. 1 ). Methanediol contains two pairs of protic and hydridic hydrogen atoms per unit resulting in two equivalents of hydrogen gas ( Fig. 1 ). Equally to formic acid all protic and hydridic hydrogens in methanediol are accessible for dehydrogenation, resulting in a weight efficiency of 8.4 wt% H 2 per molecule. Thus, FA acts as a hydride donor and water as a proton donor, which represents a FA-based molecular approach for indirect water-splitting. The dehydrogenation of methanediol probably occurs in a two-step reaction, where the methanediol is converted into formic acid under hydrogen evolution (1 st eq. H 2 ), and then the formic acid is further converted into carbon dioxide and hydrogen (2 nd eq. H 2 ). 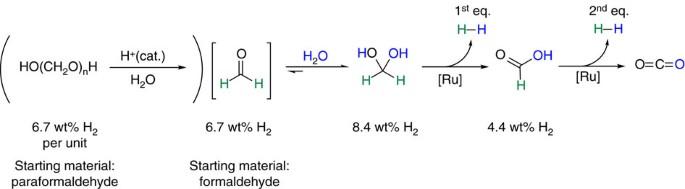Figure 1: Reaction pathway. Proposed reaction sequences using paraformaldehyde or formaldehyde as a hydride source and water as a proton source for the subsequent hydrogen generation. Figure 1: Reaction pathway. Proposed reaction sequences using paraformaldehyde or formaldehyde as a hydride source and water as a proton source for the subsequent hydrogen generation. Full size image Previous reports about formic acid and methanol showed that the presence of at least catalytic amounts of base is crucial for the successful dehydrogenation of the hydrogen carrier [8] , [15] , [16] , [18] . In contrast, we found that the dehydrogenation of methanediol derived from FA or pFA is possible also in absence of base additives ( Supplementary Fig. 2 : 37 wt%. aqueous FA solution). However, the addition of base shows some positive effect and accelerates the dehydrogenation reactions carried out at ambient pressure. The efficiency of the catalytic dehydrogenation depends on the applied temperature with the best catalyst performance at 95 °C (368 K). High hydrogen yields (84%) were already achieved within short reaction time (<60 min) and recharge of the catalyst solution was possible by adding FA or pFA to the reaction mixture. Composition of the gaseous and liquid phases Taking into account the proposed reaction sequence in Fig. 1 , the gaseous phase was monitored by means of sensitive mass spectrometry (MS) techniques (see Methods). Herewith a semiquantitative characterization of the gaseous phase composition, besides the quantification with mass-flow meters, was obtained. Indeed, the time-resolved MS analysis confirms that in the initial period the composition contains much larger amounts of hydrogen rather than carbon dioxide ( Supplementary Figs 3,4a ). It should be pointed out that neither FA nor CO is present in significant amounts in the gaseous phase as confirmed by labelling experiments with 13 C-pFA and H 2 18 O, which underlines the robustness (no FA extrusion) and the selective dehydrogenation as no relevant CO formation is observed ( Supplementary Figs 3,4a,b ; Fig. 2 ). This stays in agreement with previous studies using formic acid, where no CO formation has been observed by MS and gas chromatography analysis [8] . Note, a residual MS signal in Fig. 2 at 29 m / z can be assigned to natural 14/15 N 2 ( 14 N: 99.634% and 15 N: 0.366%) and a residual signal at 30 m / z can be assigned to NO formed under MS conditions (also present as a background signal of analysed air). The absence of FA and CO is important to guarantee high efficiency for fuel cell applications, as it is known that formic acid can decompose to CO and water at elevated temperature [36] . 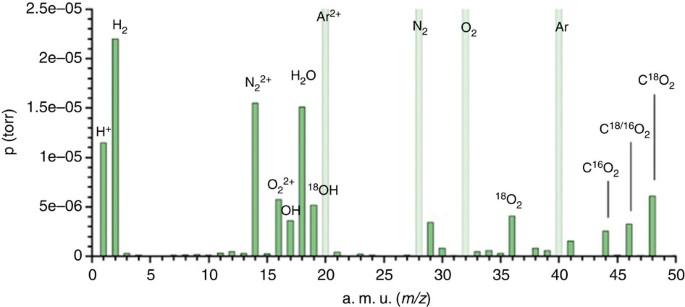Figure 2:Mass spectrogram of isotope-labellingexperiment with H218O. Gaseous phase analysis of the pFA decomposition in presence of18H2O under air with argon as the carrier gas; the peak at 18m/zmay include intensity of trace amounts of18O22+and the peak at 20m/zmay include traces of H218O+. The intensive peaks related to argon, nitrogen and oxygen are depicted as dashed bars (for full spectrogram seeSupplementary Fig. 5). Note, a residual MS signal inFig. 2at 29m/zcan be assigned tonatural14/15N2+(14N: 99.634%), (15N: 0.366%) and a residual signal at 30m/zcan be assigned to NO+formed under MS conditions (also present as background signal of analysed air). Figure 2: Mass spectrogram of isotope-labelling experiment with H 2 18 O . Gaseous phase analysis of the pFA decomposition in presence of 18 H 2 O under air with argon as the carrier gas; the peak at 18 m/z may include intensity of trace amounts of 18 O 2 2+ and the peak at 20 m/z may include traces of H 2 18 O + . The intensive peaks related to argon, nitrogen and oxygen are depicted as dashed bars (for full spectrogram see Supplementary Fig. 5 ). Note, a residual MS signal in Fig. 2 at 29 m / z can be assigned to natural 14/15 N 2 + ( 14 N: 99.634%), ( 15 N: 0.366%) and a residual signal at 30 m / z can be assigned to NO + formed under MS conditions (also present as background signal of analysed air). Full size image During the ongoing reaction, the composition of the gaseous phase changes. In the late step, the gas stream contains relatively more carbon dioxide in comparison with hydrogen than in the initial step ( Supplementary Fig. 3 ). Therefore, it is more likely that first methanediol is converted into formic acid and one equivalent of hydrogen, and then formic acid is converted into hydrogen and carbon dioxide. Indeed, the nuclear magnetic resonance (NMR) analysis of an aliquot showed that reasonable amounts of formic acid (15.6%) are formed during the course of the reaction. This indicates that the following formic acid dehydrogenation plays a major role after high conversion of methanediol into formic acid and hydrogen. To obtain further information about the dehydrogenation pathway and the composition of the gaseous phase and species in the liquid phase, the substrate scope was extended to isotope-labelled compounds such as deuterated FA in deuterium oxide ( Supplementary Table 1 ; entry 2) and pFA labelled with 2 H and 13 C. The pFA easily forms FA under slightly acidic conditions, in fact the pH of distilled water used and stored under air is acidic enough owing to the dissolved CO 2 , but a small amount of acid additive is beneficial. The solvation of [(Ru(p-cymene)) 2 ( μ- Cl) 2 Cl 2 ] 1 in water results at pH>5.0 in the formation of [(Ru(p-cymene)) 2 (μ 2 -OH) 3 ] + 2 and free chloride [37] , thus providing a sufficiently acidic condition/environment. To yield further insights on the reaction mechanism, we performed a series of experiments with non-deuterated ( Supplementary Table 1 ; entries 3–5), deuterated ( Supplementary Table 1 ; entries 7–9) and 13 C-labelled ( Supplementary Table 1 , entries 10–12) pFA with H 2 O ( Supplementary Table 1 , entries 3, 9 and 10), D 2 O ( Supplementary Table 1 , entries 4, 7 and 12), HDO ( Supplementary Table 1 , entries 5, 8 and 11) and H 2 18 O ( Supplementary Table 1 , entry 6; Fig. 2 ). The monitoring of the gaseous phase by MS and the analysis of the liquid phase by NMR and electrospray ionization (ESI)–MS give further information about the reaction pathways and the ruthenium species. The gaseous phase analysis by MS of the labelled experiments provides evidence that both water and (para)FA are the sources of the hydrogen. With (HO(CH 2 ) n H) in H 2 O hydrogen and carbon dioxide are detected in the gaseous phase ( Supplementary Table 1 , entry 3), likewise for (DO(CD 2 ) n D) in D 2 O we detected D 2 and CO 2 ( Supplementary Table 1 , entry 7). One could expect that the dehydrogenation of non-deuterated pFA (HO(CH 2 ) n H) in D 2 O results in dominating formation of HD gas, with the deuteron originating from D 2 O and the hydride from the pFA ( Supplementary Table 1 , entry 4). Interestingly, we observed the following order of formation: with highest abundance, D 2 was detected, followed by HD and then H 2 . Similar observations were made with dinuclear ruthenium carbonyl complexes for the dehydrogenation of partially deuterated formic acid HCO 2 D or DCO 2 H. Here the authors reported the initial predominant formation of H 2 , followed by HD and D 2 formation [38] . This indicates that H/D scrambling is catalysed by a ruthenium species between the D 2 O and the C–H bonds of the in situ- generated methanediol previous to the dehydrogenation to formic acid, and it proves that water acts as a source of hydrogen, as methanediol is only formed from FA in the presence of water. Note, in our experiments H/D-exchange was observed by 1 H and 2 H NMR analysis of the Ru-H and water signal (H 2 O/HDO/D 2 O). Vice versa, the experiment with deuterated pFA (DO(CD 2 ) n D) in H 2 O resulted mainly in the formation of H 2 , followed by H/D and only traces of D 2 ( Supplementary Table 1 , entry 9). The lack of D 2 in the gaseous phase can be explained, as significant amounts of D 2 O have been formed and detected, which proves the H/D scrambling between H 2 O and the C–D bonds of the in situ -formed D 2 -methanediol ( Supplementary Table 1 , entry 9). The treatment of (DO(CD 2 ) n D) with HDO shifts the formation to HD, while (HO(CH 2 ) n H) with HDO gives H 2 as main product ( Supplementary Table 1 , entries 5 and 8). The reaction with (HO( 13 CH 2 ) n H) in H 2 O, HDO or D 2 O resulted in the formation of 13 CO 2 ( Supplementary Table 1 , entries 10–12) besides the above mentioned H/D scrambling. The dehydrogenation of (HO(CH 2 ) n H) in H 2 18 O ( Supplementary Table 1 , entry 6; Fig. 2 ) results in formation of H 2 , carbon dioxide C 18 O 2 , C( 16 O 18 O) and C 16 O 2 proving the complete incorporation of one molecule of water into FA forming methanediol, including additional oxygen scrambeling giving all three 16 O/ 18 O-labelled carbon dioxide species ( Fig. 2 ). Moreover, the formation of 18 O 2 ( Fig. 2 ) indicates that water is oxidized at least partially in another reaction pathway probably involving ruthenium hydrides and hydroxo-bridged ruthenium dimers. Note, hydroxo-bridged dimers are readily formed in presence of the water [37] . Hence, this can be assigned as indirect water-splitting resulting in solely gaseous products. Furthermore, we would like to emphasize that water-splitting has not been observed in absence of a FA source. In situ characterization by NMR Analysis of the reaction mixture by one- and two-dimensional (2D) 1 H and 13 C NMR experiments provided evidence for the presence of a dinuclear ruthenium hydride [(Ru(p-cymene)) 2 μ -H( μ -HCO 2 ) μ -Cl] + 3 ( Fig. 3 ). Coupling patterns observed for the p-cymene ligand indicate asymmetric Ru centers, and integration of the 1 H NMR signals allows to conclude that the catalyst is a dinuclear mono-hydrido complex. Chemical shifts of the ligand system are in good agreement with the ones observed for similar, carboxylate complexes [39] . There is only one type of arene ligand present, which shows clearly a H,C long range correlation to the bridging hydride signal at −7.08. Another long range connectivity is observed between the bridging formate unit and the hydride. In addition, through-space couplings were detected by way of 2D H,H nuclear overhauser effect spectroscopy experiments: cross peaks revealed interactions between p-cymene ligand and hydride, as well as proximity between p-cymene and formiate ( Supplementary Figs 6–24 ; Supplementary Table 2 ). Besides the compound described above, other Ru complexes were also visible in the 1 H NMR spectrum: besides traces of [(Ru(p-cymene)) 2 ( μ -Cl) 2 Cl 2 ] 1 and its hydrolysis products, for example, [(Ru(p-cymene)) 2 ( μ -OH) 3 ] + 2 , at least one other Ru(p-cymene) complex could be identified. These three additional species are in chemical exchange, as evidenced by H,H EXchange SpectroscopY experiments, most likely exchange between chlorido and hydroxo ligands ( vide infra ) [37] , [40] . In contrast to the previously reported acetato complexes [39] , the solute dynamic formiato complex 3 with Cl − as counter ion is only stable in solution in presence of methanediol or formic acid in water, thus isolation of 3 as chloride salt was not possible ( Supplementary Figs 6 and 7 ), but we achieved the isolation as BF 4 -salt 3-BF 4 ( vide infra ). 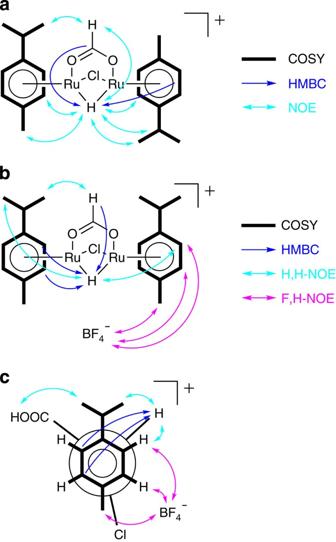Figure 3: Visualization of NMR results. Depiction of the correlated spectroscopy (COSY), nuclear overhauser effect (NOE) contacts and H,C long range correlations in (a) [(Ru(p-cymene))2μ-H(HCO2)μ-Cl]+Cl−3(in water) (b) for3-BF4(in CD2Cl2; front view) and (c) for3-BF4(in CD2Cl2; side view). Figure 3: Visualization of NMR results. Depiction of the correlated spectroscopy (COSY), nuclear overhauser effect (NOE) contacts and H,C long range correlations in ( a ) [(Ru(p-cymene)) 2 μ -H(HCO 2 ) μ -Cl] + Cl − 3 (in water) ( b ) for 3-BF 4 (in CD 2 Cl 2 ; front view) and ( c ) for 3-BF 4 (in CD 2 Cl 2 ; side view). Full size image In situ characterization by ESI–MS Further analysis of aliquots of the liquid phase of (HO(CH 2 ) n H) in H 2 O by means of ESI–MS showed that several ruthenium species are present, taking into account the isotope pattern of ruthenium ( Supplementary Table 1 ; Supplementary Figs 25 and 26 ). Only one of them incorporates a formiate-bridging ligand and it can be assigned to [(Ru(p-cymene)) 2 μ -H( μ -HCO 2 ) μ -Cl] + 3 ( vide supra ) and its isotopologues 4 – 8 ( Supplementary Table 1 ). A previous report about formic acid dehydrogenation assigned the cation as [(Ru(p-cymene)) 2 H( μ -HCO 2 )μ-Cl] + by means of ESI–MS experiments [8] . The other species are formed when [Ru(p-cymene)Cl 2 ] 2 1 is dissolved in water under slightly acidic conditions; for example, [(Ru(p-cymene)) 2 ( μ -OH) 3 ] + 2 ( vide supra ; for more examples see Supplementary Figs 25 and 26 ) [37] , [40] . In the present case, we can distinguish between ruthenium dimers bridged by combinations of formiato, hydrido, chlorido or hydroxo ligands ( Supplementary Figs 25 and 26 ). Among them, the dimeric formiate- and hydride-bridged ruthenium complex 3 can be taken into account to play a role in the methanediol dehydrogenation owing to reported activity of ruthenium dinuclear complexes in formic acid dehydrogenation [8] , [38] . The analysis of aliquots of the liquid phase of the above discussed labelling experiments allows the assignment of complexes that reacted with methanediol. The formiato-bridged ruthenium dimer shows isotope shifts when labelled with 2 H, 13 C and 18 O ( Fig. 4 ). The latter experiment proves again that water participates in the process also as a source of hydrogen via the methanediol formation and dehydrogenation. The labelled complexes clearly show the characteristic isotope shifts and stay in agreement with simulated spectrograms ( Fig. 4 ). Note, no anionic complexes were detected in the ESI(−)–MS mode. 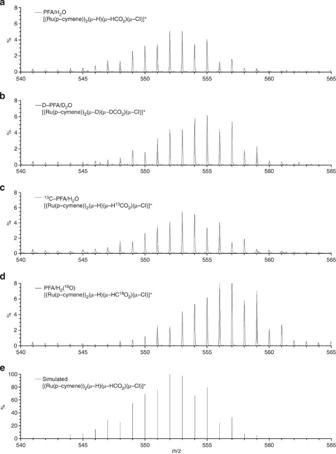Figure 4: ESI–MS spectrograms of the cations. (a) [(Ru(p-cymene))2μ-H(HCO2)μ-Cl]+3(pFA in H2O, M=553;Supplementary Table 1, entry 3), (b) [(Ru(p-cymene))2μ-D(DCO2)μ-Cl]+4(D-pFA in D2O, M=555;Supplementary Table 1, entry 7), (c) [(Ru(p-cymene))2μ-H(H13CO2)μ-Cl]+7(13C-pFA in H2O, M=554;Supplementary Table 1, entry 10), (d) [(Ru(p-cymene))2μ-H(HC18O2)μ-Cl]+6(pFA in H218O, M=557;Supplementary Table 1, entry 6) derived from the pFA and water dehydrogenation and (e) simulated MS spectrogram. Figure 4: ESI–MS spectrograms of the cations. ( a ) [(Ru(p-cymene)) 2 μ -H(HCO 2 ) μ -Cl] + 3 (pFA in H 2 O, M=553; Supplementary Table 1 , entry 3), ( b ) [(Ru(p-cymene)) 2 μ -D(DCO 2 ) μ -Cl] + 4 (D-pFA in D 2 O, M=555; Supplementary Table 1 , entry 7), ( c ) [(Ru(p-cymene)) 2 μ -H(H 13 CO 2 ) μ -Cl] + 7 ( 13 C-pFA in H 2 O, M=554; Supplementary Table 1 , entry 10), ( d ) [(Ru(p-cymene)) 2 μ -H(HC 18 O 2 ) μ -Cl] + 6 (pFA in H 2 18 O, M=557; Supplementary Table 1 , entry 6) derived from the pFA and water dehydrogenation and ( e ) simulated MS spectrogram. Full size image Catalyst performance and isolation Regarding the catalytic activity, we have strong evidence that complex 3 is an active species as indicated by NMR analysis and isotope-labelling experiments. Moreover, we found that metal nanoparticles are unlikely to be active for this reaction under these conditions, as control experiments with nanoparticles and supported metal catalysts showed no activity. Taking into account the identified dinuclear ruthenium species [(Ru(p-cymene)) 2 μ -H( μ -HCO 2 ) μ -Cl] + 3 by NMR, ESI–MS and the gaseous composition by MS gas analysis, we envision that the catalytic process for methanediol dehydrogenation is similar to the reported formic acid dehydrogenation by dinuclear ruthenium complexes [38] . Regarding the optimization of the catalytic performance of the simultaneous FA dehydrogenation and water-splitting via methanediol, we considered the application of a pH buffer (K 3 PO 4 ), varied the catalyst loadings ( Supplementary Fig. 2 ), FA concentration and temperature. Practical catalyst precursor loadings can be as low as 0.1 mol% with the best performance at 95 °C (368 K). The application of a pH buffer seems to be beneficial, as we found that in absence of a pH buffer the solution becomes strongly acidic and with the increasing acidity the reaction rate drops. However, the conversions are stable between pH 2.4 (75%) and pH 9 (73%) with a maximum at pH 5.5 (85%) and dropped to 53% at pH 1.4. Therefore, a pH buffer is beneficial but not crucial, and makes the catalytic system applicable for a wide pH range of aqueous systems containing FA. Moreover, under basic conditions the gas flow becomes very intensive in the initial reaction period, therefore lower catalyst loadings (<0.14 mol%) can be used, respectively large FA loadings in diluted solution are more feasible for a controlled low flow of hydrogen. Good performance for recycling experiments and long-term stability could be achieved with both aqueous FA or pFA in water as a hydrogen source. It was possible to obtain a continuous hydrogen production by simply recharging the aqueous phase with pFA (three times). Also, with large substrate loadings of aqueous FA, we obtained a stable gas flow over 2 days even at 65 °C. Since simultaneously water is consumed for the generation of the methanediol, after prolonged time water as fuel must be added as well. For proving the role of complex 3 in the FA-assisted water-splitting, we succeeded to isolate the complex from the ongoing catalytic process as its BF 4 -salt ( 3-BF 4 ). Also we synthesized complex 3-BF 4 by treatment of complex 1 with formic acid. The NMR ( Supplementary Figs 14–24 ; Supplementary Table 3 ) and ESI–MS data of the cationic complexes 3 and 3-BF 4 are in full agreement with each other. With the independently synthesized compound, which yielded NMR spectra ( Supplementary Figs 14–24 ) that are in complete accordance with the ones obtained from the isolated complex, further characterization was obtained by diffusion and nuclear overhauser effect (NOE) NMR experiments ( Supplementary Figs 14–24 ). Thus, for the 3-BF 4 complex, ion pairing and a site-specific coordination of the counter ion could be detected (for details see SI and Supplementary Figs 14–24 ). Consequently, we used the synthesized complex 3-BF 4 for the FA-assisted water-splitting and it revealed also high activity similar to the in situ system with complex 1 . The pure gaseous stream solely containing hydrogen and carbon dioxide resulting from the catalytic conversion of aqueous FA and pFA, respectively, methanediol, makes this proof of concept interesting for all types of hydrogen fuel cells using water and a liquid organic hydrogen carrier. In particular, the tuneable flow rate and easily separable gas mixture allows the application in engines, overcoming technical difficulties with pressure cylinders. The application of such air-stable catalysts may overcome drawbacks related to inert gas techniques. FA and pFA are prepared industrially by silver or metal oxide-catalysed dehydrogenation of methanol (Formox process). Methanol itself is accessible from carbon monoxide, from renewable sources [41] , or via carbon dioxide hydrogenation [19] . Therefore, an envisioned CO 2 neutral approach would be to complete the circuit of our presented system by including the extruded CO 2 through hydrogenation into methanol (ref. 19 ), which can be subsequently oxidized to FA or pFA via the Formox process, note that partial reduction of CO 2 to FA is an unresolved issue ( Fig. 5 ). 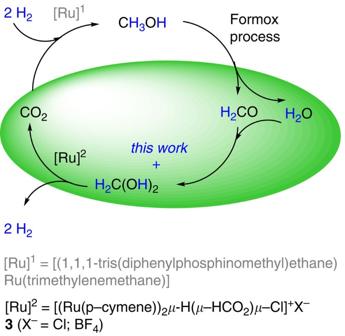Figure 5: Hydrogen storage cycle. A full cycle for a CO2-based hydrogen storage system including catalysts3or3-BF4. Figure 5: Hydrogen storage cycle. A full cycle for a CO 2 -based hydrogen storage system including catalysts 3 or 3-BF 4 . Full size image For mobile H 2 -fuelled devices, the CO 2 capturing and the regeneration of the FA from CO 2 might be decoupled from the fuel cell system. CO 2 capturing and its hydrogenation is more suitable to be performed at industrial plants using CO 2 -containing exhaust gas streams rather than an on-board regeneration of the spent fuel. However, there are still some obstacles for future research regarding the straight forward conversion of carbon dioxide into FA, as until now FA is only accessible from methanol oxidation in a practical way. The homogeneous-catalysed dehydrogenation of aqueous FA and pFA solutions in our present work show a robust and air-stable method for hydrogen production at low temperature, mild conditions and tuneable rates. Previous limitations of homogeneous systems using formic acid or methanol as a hydrogen storage material, such as low weight efficiency (formic acid), application of air-sensitive catalysts (methanol) or gaseous side-products (CO) have been avoided. However, this approach is still limited to pFA or technical grade aqueous FA (37 wt%) giving a H 2 weight efficiency of about 5 wt%, although methanediol has a hydrogen content of 8.4 wt%. For this reason future studies will include the optimization to push the weight efficiency of this approach to its limit above 8 wt% to make it more attractive for potential application. Although the catalyst is active in basic and acidic solution, the pH value has to be taken into account for best catalytic activity, and this must be considered for tailoring the performance of future catalysts and overcome limitations in application. Furthermore, this approach might be suitable for simultaneous hydrogen production and decontamination of industrial wastewater with FA impurities—a waste-to-value approach. The latter aspect could be of interest as FA contamination of wastewater remains a worldwide problem to be solved, since it might be a step forward to overcome these obstacles. General considerations pFA was purchased from Alfa Aesar . pFA-D 2 , hydrogenoxide- 18 O, D 2 -FA solution (20 wt% FA in D 2 O), non-deuterated FA (37 wt% FA in H 2 O) and [RuCl 2 ( p -cymene)] 2 were purchased from Sigma Aldrich. pFA- 13 C was purchased from Cambridge Isotope Laboratories. All chemicals were used without further purification. If not mentioned separately, deionized water was used for all experiments. The catalytic reactions, catalyst isolation and catalyst syntheses were usually performed at least three times. All dehydrogenation reactions were carried out without precautions against moisture or oxygen unless otherwise stated. All dehydrogenation data were corrected by experimental data of empty glass reactors at the set temperature to compensate for thermal expansion. The amount of released gas was determined with a mass flow meter of the manufacturer MKS connected via an analogue connection to a desktop computer. MS investigations (gas composition) in the gas phase were conducted with a HPR-20 gas analysis system by Hiden Analytical and were directly connected to the catalysis setup ( Supplementary Fig. 28 ). The HPR-20 QIC (Hiden Analytical) has a MS detection limit <0.09 p.p.m. as xenon in air is detectable. Note the MS has sensitivity down to partial pressures of 10 −10 torr (note: spectrometer-specific unit is torr not MPa). The data were recorded with the software RealView 3.0 by ABACOM. Data processing was conducted with QtiPlot-0.9.9 (Ion Vasilief). Characterization and physical measurements 1 H, 2 H and 13 C NMR spectra were recorded on Bruker Avance 400 MHz, Bruker Avance 300 MHz, Bruker Avance III 500 MHz or Bruker Avance II + 600 MHz spectrometers. 1 H, 19 F, 11 B and 13 C NMR chemical shifts are reported in p.p.m. NMR data are presented as follows: chemical shift, multiplicity (s, singlet; d, doublet; t, triplet; q, quadruplet; m, multiplet and/or multiple resonances), coupling constants are given in Hertz (Hz), relative signal intensities ( 1 H) were obtained by integration. All NMR signals were assigned on the basis of 1 H and 13 C( 1 H), gradient-edited H-H correlated spectroscopy, H-H nuclear overhauser effect spectroscopy, H-C heteronuclear multiple-quantum correlation and H-C heteronuclear multiple bond correlation experiments. Water and FA signals were suppressed by standard solvent suppression sequences. Spectra were recorded at 298 K if not otherwise indicated. NMR samples of complex 3 were prepared by dissolving 20 mg (0.03 mmol) of [RuCl 2 (p-cymene)] 2 and 7–8 mg pFA with 675 μl H 2 O or D 2 O in a gas chromatography vial equipped with a magnetic stirring bar. After addition of 1 μl of 1M aqueous H 2 SO 4 solution, the sample was stirred at 95 °C (368 K) for 35 min. The mixture was cooled to room temperature and transferred to a 5-mm NMR tube. In case of H 2 O solutions, an insert containing 100 μl of D 2 O was introduced to lock the sample for NMR measurements. The 2D H-F HOESY experiments were performed with the isolated/synthesized complex 3 -BF 4 analysed in CD 2 Cl 2 . HOESY experiments were acquired using a gradient-selected version [42] . Semiquantitative spectra were acquired using a 3.5-s relaxation delay and 700-ms mixing time. For the determination of self-diffusion coefficients, 1 H- and 19 F-PGSE NMR experiments were carried out for 3-BF 4 in CD 2 Cl 2 at 298 K for cation ( 1 H) and anion ( 19 F). Measurements were performed by using a stimulated echo pulse sequence with LED implemented [43] on a Bruker Avance 400 MHz spectrometer equipped with a GAB gradient amplifier and a triple resonance broad band inversed (TBI) probe with a Z-gradient coil. The diffusion coefficients for complex 3-BF 4 (cation D =4.1*10 −9 m 2 s −1 and anion D =4.8*10 −9 m 2 s −1 ) indicate together with strong NOE contacts observable from H,F HOESY spectra the presence of ion pairing. A small portion of the NMR solution was also used for ESI–MS experiments ( vide infra ): for this purpose, the sample was further diluted to a concentration of 1 mg ml −1 . From this stock solution one drop was diluted in 1.5 ml H 2 O or D 2 O; the sample with H 2 18 O was diluted with acetonitrile to avoid oxygen scrambeling with H 2 O. ESI–MS investigations were performed on a LTQ XL Thermo Scientific. Dehydrogenation of neat aqueous FA solutions Exemplary experiment: 12.9 μmol (0.1 mol%) [RuCl 2 ( p -cymene)] 2 1 were added to 13.55 mmol of an aqueous FA solution (37 wt% FA) into a small round-bottomed flask, the flask was connected to the measuring setup. The reaction mixture was heated to 95 °C (368 K) yielding 300 ml gas (H 2 /CO 2 ) in 200 min for complex 1 . The same protocol has been used applying [(Ru(p-cymene)) 2 μ -H( μ -HCO 2 ) μ -Cl] + BF 4 − 3-BF 4 as a catalyst yielding 340 ml gas (with a K 3 PO 4 pH buffer) and 180 ml after 200 min under base-free conditions. Dehydrogenation of aqueous FA solutions Exemplary experiment: 18.1 μmol (0.14 mol%) [RuCl 2 ( p -cymene)] 2 were added with 1.9 ml water and 13.55 mmol of an aqueous FA solution (37 wt% FA) into a small round-bottomed flask. After 0.21 mmol (44.6 mg) K 3 PO 4 were added to the content, the flask was connected to the measuring setup. The reaction mixture was heated to 95 °C (368 K) giving 25% conversion (TON=188) already after 67 min. Dehydrogenation of pFA in water (example) Exemplary experiment: 0.13 mmol [RuCl 2 ( p -cymene)] 2 were added with 2.7 ml water and 1.0 mmol pFA into a small round-bottomed flask. After 5.2 μmol (5.2 μl) of 1M H 2 SO 4 (aqueous) were added to the content, the flask was connected to the measuring setup. The reaction mixture was heated to 95 °C (368 K) for 74 min giving 75% conversion. Isolation of complex 3-BF 4 [RuCl 2 ( p -cymene)] 2 1 (0.13 mmol (80 mg)) and 1 mmol (30.0 mg) pFA were suspended in 2.5 ml water. The mixture was heated to 95 °C (368 K) and stirred for 45 min. The solution was cooled down to room temperature and filtered. NaBF 4 (0.13 mmol (14.3 mg)) were added to the filtrate and stirred for 2 min. The precipitate was filtered off, washed two times with 0.5 ml water and dried under reduced pressure, the solid material was analysed by NMR staying in full agreement with the data obtained for the cation of complex 3 . Melting point: 164–166 °C (437–439 K) (decomposition); 1 H NMR (300 MHz, CD 2 Cl 2 ): δ 6.83 (d, J =0.8 Hz, 1H), 6.51 (d, J =5.9 Hz, 1H), 6.17 (d, J =6.1 Hz, 1H), 5.79 (d, J =6.0 Hz, 1H), 5.44 (d, J =5.9 Hz, 1H), 2.70 (hept, J =6.9 Hz, 1H), 2.12 (s, 3H), 1.31 (d, J =6.9 Hz, 3H), 1.30 (d, 6.9 Hz, 3H), −7.26 (s, 1H); 13 C NMR (75 MHz, CD 2 Cl 2 ): δ 174.9, 104.6, 97.8, 86.2, 84.3, 80.9, 78.8, 31.6, 22.7, 21.8, 19.2; 19 F NMR (282 MHz, CD 2 Cl 2 ): δ −152.0 (q, J =1.1 Hz); 11 B NMR (282 MHz, CD 2 Cl 2 ): δ −0.9 (quin, J =1.1 Hz); HRMS ( m / z ): [M] + calcd. for C 21 ClH 30 O 2 Ru 2 , 553.0016; found, 553.0018 (see Supplementary Fig. 27 ). Synthesis of complex 3-BF4 using formic acid A round-bottom flask was charged with 0.65 mmol (400 mg) [RuCl 2 ( p -cymene)] 2 1 and 20 ml water. Formic acid (1.5 mmol (57 μl)) was added and the mixture was heated to 95 °C (368 K) for 15 min. The solution was quickly cooled down to room temperature and 0.65 mmol (71.4 mg) NaBF 4 was added. The precipitate was filtered off, washed two times with 1.5 ml water and dried in vacuo yielding 180 mg (0.28 mmol) 3-BF 4 ( μ -chloro,-μ-formiato, μ -hydrido( p -cymene)ruthenium(II) dimer tetrafluoroborate salt) as orange-red powder, the solid material was analysed by NMR and ESI–MS staying in full agreement with the data obtained for the complex 3-BF 4 as isolated using the procedure for isolation of complex 3-BF 4 . How to cite this article: Heim, L.E. et al. Selective and mild hydrogen production using water and formaldehyde. Nat. Commun. 5:3621 doi: 10.1038/ncomms4621 (2014).